Magneto-optical properties of trions in non-blinking charged nanocrystals reveal an acoustic phonon bottleneck Charged quantum dots provide an important platform for a range of emerging quantum technologies. Colloidal quantum dots in particular offer unique advantages for such applications (facile synthesis, manipulation and compatibility with a wide range of environments), especially if stable charged states can be harnessed in these materials. Here we engineer the CdSe nanocrystal core and shell structure to efficiently ionize at cryogenic temperatures, resulting in trion emission with a single sharp zero-phonon line and a mono exponential decay. Magneto-optical spectroscopy enables direct determination of electron and hole g -factors. Spin relaxation is observed in high fields, enabling unambiguous identification of the trion charge. Importantly, we show that spin flips are completely inhibited for Zeeman splittings below the low-energy bound for confined acoustic phonons. This reveals a characteristic unique to colloidal quantum dots that will promote the use of these versatile materials in challenging quantum technological applications. The excited state of singly charged semiconductor quantum dots (trion state) is one of the most useful states in nano-scale materials [1] , [2] , [3] , [4] . This state can provide many prototypical quantum optical systems, such as two-level systems, which are useful for single-photon sources [1] , [2] , and three-level systems useful for coherent control applications [3] . It also offers complete optical control and readout of the spin of a single charge [4] , useful for quantum information processes. The use of colloidal nanocrystals (NCs) in such applications is still nascent, despite their rapidly maturing technology and their wide compatibility with different photonic technologies and environments [5] . Charged NCs serve as the ideal system for investigating charge-carrier spin properties. To date, such properties have only been indirectly investigated in CdSe NC ensembles [6] , [7] yielding results that could not be reconciled with theoretical estimates [8] . In a charged NC, both the ground state and the band-edge excited state have an angular momentum determined by a single-charge carrier. Therefore, it is possible to directly measure both the electron and hole g -factors using magneto-optical spectroscopy, gaining access to information on spin relaxation. This latter property has special relevance for colloidal NCs, where their finite size (usually less than 10 nm) results in discrete phonon modes [9] , [10] with a well-defined minimum energy (that is, the maximum phonon wavelength must be smaller than the NC size) [11] . At low temperatures, as long-wave acoustic phonon modes cannot develop, relaxation between states with energy separations smaller than the lowest phonon energy should be inhibited, giving rise to an ‘acoustic phonon bottleneck’ [12] . In contrast, widely studied self-assembled quantum dots have a quasi-continuous acoustic phonon spectrum that contributes to phonon-mediated spin relaxation [13] , [14] . The potential benefit of an acoustic phonon bottleneck would be the ability to operate quantum spin technologies with high external fields suitable for aligning and freezing random environmental spins (for example, nuclear spins or magnetic defects) that otherwise cause spin decoherence [15] . Thus, confined acoustic phonon modes in NCs could ultimately provide a decoherence-free subspace for spin states, if this property can be harnessed. Spin relaxation in colloidal NCs has been a subject of recent interest that has so far been focused solely on neutral NCs with spin relaxation inferred from detailed knowledge of the band-edge exciton fine structure. A series of ensemble measurements using polarization-resolved heterodyned transient grating spectroscopy has uncovered a range of different spin relaxation processes at room temperature, indicating spin relaxation occurs on sub-picosecond time scales [16] , [17] . Conversely, at cryogenic temperatures, single-NC spectroscopy has revealed spin relaxation times between the lowest bright and dark states extended into the nanosecond time scale [18] , [19] , [20] . However, in these cases, the energy difference between the exciton fine structure states is of the order of acoustic phonon energies in the system. In addition, spin relaxation between these states involves two spins (electron and hole), which complicates the interaction. In comparison, spin flips between trion states involve only a single charge, which considerably simplifies the system. Although prospective trion properties in NCs bode well for quantum applications, reports of emission from charged CdSe NCs [19] , [21] , [22] , [23] , [24] , [25] indicate that it is either inefficient at room temperature or unstable (because the NCs randomly switch between the neutral and charged state). Stable trion emission has been reported at low temperatures, however, NCs exhibiting this emission were rare [24] . In addition, spectroscopic identification of the trion charge was tentative [19] , [24] , relying on conflicting numerical simulations [26] , [27] . In all cases, the reported trion emission was incidental. Measurements of NCs designed to reliably remain charged and exhibit stable bright trion emission have not yet been reported. In this article, we use an engineered synthesis of CdSe NCs with core and shell properties designed to promote efficient photo-charging and stable trion emission at cryogenic temperatures. Dispersion of the NCs aspect ratio leads to trion emission covering a wide range of heavy-hole and light-hole mixing. We use magneto-optical spectroscopy to directly measure the electron and hole g -factors, for the first time. Relaxation of the trion spin identifies the trion charge. Spin relaxation is found to sensitively dependent on the magnitude of the Zeeman splitting, the onset of which displays a well-defined threshold; the signature of an acoustic phonon bottleneck. Engineering trion emission We synthesize CdSe/CdS 4 /ZnS 1 core/shell/shell NCs to promote stable and efficient trion emission at cryogenic temperatures. A large NC core is used to minimize Auger effects [28] , a CdS shell promotes electron access to the NC surface [23] , [29] , [30] ( Fig. 1a ) and a thin ZnS shell improves chemical stability. A CdSe zinc-blende crystal structure was chosen to allow investigations of NCs with varying heavy-hole and light-hole influence ( Fig. 1b ). The exciton fine structure is calculated for a 5.4-nm width core (matching that determined from the synthesis sizing calibration), across an aspect ratio range determined by TEM (transmission electron microscope) analysis. The predicted energies closely match those found with these NCs, indicating that the core size predominantly defines the fine structure splitting in these nanoheterostructures. The synthesized NCs are easily photo-charged, (that is, they readily eject a charge carrier when excited above the band-edge using a 532 nm laser) resulting in efficient trion emission at cryogenic temperatures. An example of single-NC photo-charging (transitioning from neutral to trion emission) is shown in Fig. 1d . We categorize two trions with different binding energies: ~20 meV for 90% of the NCs and ~2 meV for the remaining. The quality of single-NC trion emission is demonstrated by long periods of blink-free shot noise-limited emission ( Fig. 1e ) that can continue for hours. Trion QYs close to unity are indicated by an unvarying count rate for both neutral and trion emission in the weak pump regime as shown in Fig. 1d . Photon-correlation measurements under pulsed excitation ( Fig. 1f ) show that the charged biexciton is highly efficient (~80%) indicating that the emission from both trion charge species is efficient [31] . This suggests that the main NC ionization pathway is not Auger assisted [28] , but most likely a tunnelling process and hence dependent on the shell and surface properties. 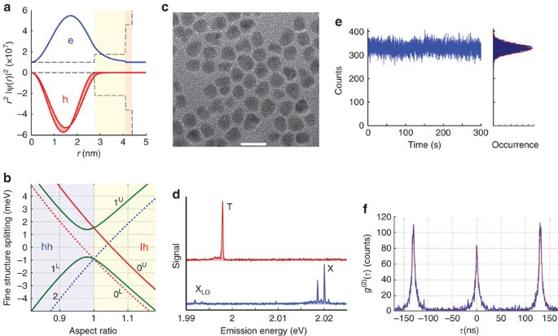Figure 1: Designing CdSe NCs for efficient trion emission. (a) Radial electron and hole wavefunctions (heavy hole hh and light hole lh) for a 5.25 nm spherical CdSe core with a two-part shell consisting of four monolayers of CdS and one monolayer of ZnS. The relative confinement potentials are also indicated (dashed). (b) The band-edge fine structure calculated for a CdSe NC with a 5.4 nm zinc-blende core verses aspect ratio (for ellipsoidal perturbations). The angular momentum of the states is indicated in the figure. Dark states are indicated by dotted lines. (c) TEM image of the CdSe/CdS4/ZnS1NCs with an approximately spherical shape with a mean diameter of 10 nm (scale bar, 20 nm). (d) Single-NC spectra before (X) and after (T) photo-charging. The accumulated photocounts for each spectrum are equivalent, indicating unity quantum yield of the trion (obtained at 2 K and 125 W cm−2pump irradiance). (e) Typical time trace of trion emission obtained from a single NC (50 ms time resolution) at 2 K showing blink-free shot noise-limited emission over 5 min. The red dashed curve is the Poisson distribution calculated using the mean counts per time bin. (f)g(2)(τ) measurement of a single-NC trion emission under pulsed emission at 570 nm and 20 K. A pulse irradiance of 68 μJ cm−2corresponds to a mean number of excitations per pulse of ‹N›≈0.1. The fit is a sum of three two-sided exponentials corresponding to a trion lifetime of 4.8 ns. Figure 1: Designing CdSe NCs for efficient trion emission. ( a ) Radial electron and hole wavefunctions (heavy hole hh and light hole lh) for a 5.25 nm spherical CdSe core with a two-part shell consisting of four monolayers of CdS and one monolayer of ZnS. The relative confinement potentials are also indicated (dashed). ( b ) The band-edge fine structure calculated for a CdSe NC with a 5.4 nm zinc-blende core verses aspect ratio (for ellipsoidal perturbations). The angular momentum of the states is indicated in the figure. Dark states are indicated by dotted lines. ( c ) TEM image of the CdSe/CdS 4 /ZnS 1 NCs with an approximately spherical shape with a mean diameter of 10 nm (scale bar, 20 nm). ( d ) Single-NC spectra before (X) and after (T) photo-charging. The accumulated photocounts for each spectrum are equivalent, indicating unity quantum yield of the trion (obtained at 2 K and 125 W cm −2 pump irradiance). ( e ) Typical time trace of trion emission obtained from a single NC (50 ms time resolution) at 2 K showing blink-free shot noise-limited emission over 5 min. The red dashed curve is the Poisson distribution calculated using the mean counts per time bin. ( f ) g (2) ( τ ) measurement of a single-NC trion emission under pulsed emission at 570 nm and 20 K. A pulse irradiance of 68 μJ cm −2 corresponds to a mean number of excitations per pulse of ‹ N ›≈0.1. The fit is a sum of three two-sided exponentials corresponding to a trion lifetime of 4.8 ns. Full size image Heavy-hole and light-hole spectra Magneto-optical spectroscopy conclusively identifies the trion emission, as the absence of the electron–hole exchange interaction leads to the symmetric Zeeman splitting of a single spectral line into either two, three or four spectral lines [32] . In Fig. 2a–d , we show spectra of four different trions obtained under a 7 T magnetic field, which reveal an evolution from four peaks towards three peaks. Before photo-charging, we could characterize the neutral emission [18] , [19] , [20] of three of these NCs ( Fig. 2e–g ) where the hole band-edge state (heavy hole, light hole) was identified by the angular momentum of the lowest energy excitonic state [33] . The three-peak trion of Fig. 2a is associated with a light hole where the lowest energy exciton state, 0 L , is dark and only appears with the application of a magnetic field [33] . The four-peak spectra of trions in Fig. 2b correspond to a ‘cross-over’ regime of strong heavy-hole/light-hole mixing [33] . The last four-peak trion of Fig. 2d with depressed central peaks is consistent with a heavy-hole regime [34] . Electron and hole g -factors are determined by measuring the peak positions of the split trions ( Fig. 2h ). The data comprise g -factors determined from four-peak, three-peak and two-peak spectra. The electron g -factor is expected to be nearly isotropic [34] , which we associate with the minimal spread of the g 2 values indicating a single electron g -factor between 1.4 and 1.5. The hole g -factor (given by g 1 values), on the other hand, is spread between 0 and 1.9. 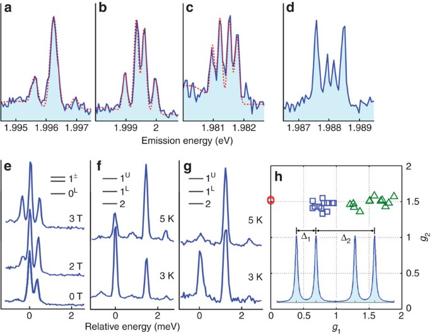Figure 2: Splitting of the trion line at 7 T. (a–d) Trion spectra from four individual NCs. (a),(b) and (c) have associated neutral spectra (e), (f) and (g), respectively. The neutral spectra are assigned according to the spectroscopic identifications previously reported in ref.33. The four-peaked spectra are consistent with heavy hole (right) or mixed heavy-hole/light-hole trions (according to the neutral spectra). The three-peaked splitting is matched to the light-hole trion due to the neutral exhibiting a lowest energy 0Ldark state33. (h) Splitting energies obtained from 27 NCs and expressed asg-factors according togi=Δi/μBB,μBis the Bohr magneton and the applied magnetic fieldB=7T. The data are characterized by NCs that split into two peaks (circles), three peaks (triangles) and four peaks (squares). The measurement protocol is depicted in the inset diagram. Note the error in each measurement is approximated by the size of the markers. Figure 2: Splitting of the trion line at 7 T. ( a – d ) Trion spectra from four individual NCs. ( a ),( b ) and ( c ) have associated neutral spectra ( e ), ( f ) and ( g ), respectively. The neutral spectra are assigned according to the spectroscopic identifications previously reported in ref. 33 . The four-peaked spectra are consistent with heavy hole (right) or mixed heavy-hole/light-hole trions (according to the neutral spectra). The three-peaked splitting is matched to the light-hole trion due to the neutral exhibiting a lowest energy 0 L dark state [33] . ( h ) Splitting energies obtained from 27 NCs and expressed as g -factors according to g i =Δ i /μ B B , μ B is the Bohr magneton and the applied magnetic field B =7T. The data are characterized by NCs that split into two peaks (circles), three peaks (triangles) and four peaks (squares). The measurement protocol is depicted in the inset diagram. Note the error in each measurement is approximated by the size of the markers. Full size image The anisotropy in the hole g -factors can be understood in terms of the underlying valence band states, which are constructed from Bloch functions associated with p -like bonding orbitals and hence are threefold degenerate. The degeneracy is lifted by the NC shape anisotropy in the case of zinc-blende NCs, hence we expect the anisotropy of the hole g -factors to be associated with the shape of the NC and therefore the magnitude of the g -factors can have an orientation dependence. The wide variation of hole g -factors plotted in Fig. 2h is consistent with anisotropic hole wavefunctions [35] . Using the spectroscopic assignments of the neutral state [33] (as shown in Fig. 2e–g ), we can assign the various spectra to different aspect ratio regions. The red circles in Fig. 2h are consistent with oblate NCs, which are dominated by heavy holes. In this case, a g -factor of 0 is predicted when a crystallographic axis is perpendicular to the magnetic field [8] . The blue squares correspond to NCs, which split into four peaks and reveal hole g -factors tightly clustered around a value of 0.75. These g -factors are associated with predominately spherical zinc-blende NCs, which places them in the regime of maximal heavy-hole/light-hole mixing where the hole wavefunction becomes approximately isotropic. Finally, the data from three-peaked trions originate from prolate NCs, which are increasingly dominated by light-hole properties and thus should be more dispersed [8] . Overall, our measurements provide a direct route to determining single-charge g -factors, which now enables unambiguous assignment of g -factors extracted from indirect ensemble measurements [6] , [7] . Trion charge assignment Asymmetry in the peak heights of the trion Zeeman spectra arises from spin relaxation in the excited state. Observation of symmetric Zeeman spectra indicates spin relaxation is much slower than the trion lifetime (Discussion). Otherwise the asymmetry of the two inner peaks resulting from significant spin relaxation will depend on the trion charge and relative g -factor magnitudes. For 4-peak spectra, g e > g h (squares in Fig. 2h ), the asymmetry of the inner peaks can identify the trion charge ( Fig. 3a ). In Fig. 3c , we show two examples of four-peak trion lines at 7 T. Among the ~100 NCs we have analysed, 3 NCs had an asymmetry associated with positive trions ( Fig. 3c ) and 7 NCs displayed the asymmetry associated with negative trions ( Fig. 3d ). All spectra that exhibited a small binding energy displayed the asymmetry of a negative trion and conversely all spectra that displayed the asymmetry of a positive trion exhibited a large binding energy. We note that most of the trions with large binding energy (positive trions) show no visible peak height asymmetry, indicating that the electron spin relaxation is likely to be slow in these systems. On the contrary, all negative trions exhibit clear peak height asymmetries, indicating that hole spin relaxation is more efficient. As 90% of the NCs display large trion-binding energies, charge identification indicates that electron ejection is the dominant ionization path in these NCs, validating our design criterion. Indeed, it has been shown that holes are predominantly trapped in interfacial defects [36] , which should be rare in NCs with good crystal quality. For our core/shell/shell NCs, CdS provides only ~4% lattice mismatch with CdSe, which facilitates good epitaxial continuation of the crystal structure [37] , [38] . Although boundary strain may cause slight energy shifts [38] , the high quantum yield of these NCs is indicative of a continuous crystal structure [37] , precluding the presence of dangling bonds that can trap a charge carrier. As the hole is predominantly confined within the CdSe core, the lack of hole traps at the core/shell interface can explain the low occurrence of negative trions in our NCs. 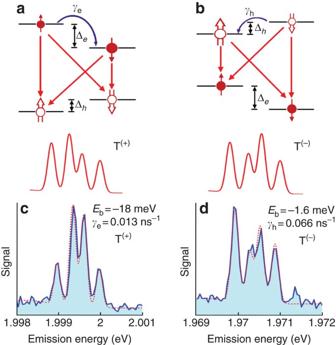Figure 3: Identification of trion charge (a) Relaxation scheme for a positive trion with Landé factorsge>ghand resultant anisotropic spectrum below. (b) Relaxation scheme for a negative trion withge>gh.and resultant anisotropic spectrum below. (c) An anisotropic four-peak spectrum from a positive trion. (d) An anisotropic four-peak spectrum from a negative trion. Corresponding binding energies,Eband spin-flip rates,γare indicated. Figure 3: Identification of trion charge ( a ) Relaxation scheme for a positive trion with Landé factors g e >g h and resultant anisotropic spectrum below. ( b ) Relaxation scheme for a negative trion with g e >g h. and resultant anisotropic spectrum below. ( c ) An anisotropic four-peak spectrum from a positive trion. ( d ) An anisotropic four-peak spectrum from a negative trion. Corresponding binding energies, E b and spin-flip rates, γ are indicated. Full size image An acoustic phonon bottleneck Acoustic phonon-mediated spin relaxation should be strongly influenced by the discrete phonon-mode spectrum, which has a low-energy bound imposed by the size of the NCs (total diameter ~10 nm). In the trion spectrum of Fig. 4a , the first acoustic phonon line is clearly resolved at an energy 650 μeV below the trion zero-phonon line. Using an average longitudinal sound velocity for the core/shell composite material, we estimate the lowest l =2 acoustic phonon energy as 600 μeV for a 10-nm NC, which is close to the observed phonon line. In addition, we resolve two more acoustic phonon peaks, including a dominant peak, which is generally attributed to the l =0 breathing mode [9] , [10] . The relative positions of the phonon peaks confirm the previous assignment (Methods), avoiding size-dependent material properties [39] . 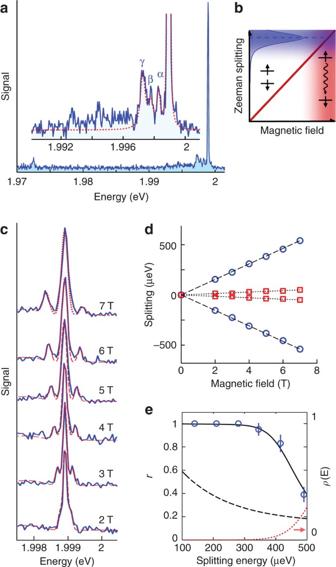Figure 4: An acoustic phonon bottleneck (a) Trion spectrum at 2 K and 0 T obtained with a 125 W cm−2, revealing the lowest energyl=2 acoustic phonon replica (α), the second orderl=2 mode (β) and the radial breathing mode (γ). (b) Illustration of the acoustic phonon bottleneck effect. Zeeman splitting as a function of magnetic field. Spin relaxation commences (red shaded region) for Zeeman splittings approaching the first acoustic phonon-mode energy (blue shaded region). An acoustic phonon bottleneck inhibits spin relaxation in the unshaded region inside the graph. (c) Splitting of the trion line with increasing magnetic field (fitting is used to determine the peak positions – dashed). (d) The peak positions determined by fitting the spectra in panelc. Note the error in each measurement, ±20 μeV, is approximated by the size of the markers. (e) Relative population of the higher energy spin state,r, as a function of the splitting energy. A fit to the data (solid line) is provided using a thermal-mixing model with a density of states,ρ(E).Theρ(E)function, shown by the red dotted curve, is a Voigt profile centred at the position of the lowest energy acoustic phonon mode (650 μeV) with a width of ~120 μeV. The expected behaviour for a constant spin relaxation rate is also indicated (dashed line). Figure 4: An acoustic phonon bottleneck ( a ) Trion spectrum at 2 K and 0 T obtained with a 125 W cm −2 , revealing the lowest energy l =2 acoustic phonon replica (α), the second order l =2 mode (β) and the radial breathing mode (γ). ( b ) Illustration of the acoustic phonon bottleneck effect. Zeeman splitting as a function of magnetic field. Spin relaxation commences (red shaded region) for Zeeman splittings approaching the first acoustic phonon-mode energy (blue shaded region). An acoustic phonon bottleneck inhibits spin relaxation in the unshaded region inside the graph. ( c ) Splitting of the trion line with increasing magnetic field (fitting is used to determine the peak positions – dashed). ( d ) The peak positions determined by fitting the spectra in panel c . Note the error in each measurement, ±20 μeV, is approximated by the size of the markers. ( e ) Relative population of the higher energy spin state, r , as a function of the splitting energy. A fit to the data (solid line) is provided using a thermal-mixing model with a density of states, ρ(E). The ρ(E) function, shown by the red dotted curve, is a Voigt profile centred at the position of the lowest energy acoustic phonon mode (650 μeV) with a width of ~120 μeV. The expected behaviour for a constant spin relaxation rate is also indicated (dashed line). Full size image Spin relaxation should depend on the magnitude of the applied magnetic field, as the lowest energy l =2 phonon-mode energy is comparable to the Zeeman splitting found at 7 T. For small Zeeman splittings, relaxation between the two spin states via the emission of a single acoustic phonon would violate energy conservation ( Fig. 4b ), which represents the acoustic phonon bottleneck. In Fig. 4c , we show an example of a trion spectrum splitting with increasing magnetic field. The peak positions found from fitting the spectra are plotted in Fig. 4d , revealing four trion transitions. Noticeably, at fields below 6 T, the spectra appear symmetric, with a peak height asymmetry marking the onset of spin relaxation. In Fig. 4e , we plot the ratio of the higher energy to lower energy side-peak heights, r , as a function of the splitting energy. As these two side transitions have the same emission rates and the same polarization, r is simply the ratio of the two excited state spin populations. Up to a splitting of 300 μeV, the two populations are approximately equal, indicating a spin relaxation time longer than the trion lifetime. An upper bound for the spin decay rate determined by the precision for estimating r (~5%) is ~0.005 ns −1 . Above 300 μeV spin relaxation increases quickly to a rate comparable to the trion recombination rate (~0.25 ns −1 ). We fit the data with a thermal-mixing model [18] , [19] that includes a spontaneous decay rate that depends on a phonon density of states, (as given by Fermi’s golden rule), where the product, ρ ( E ) γ 0 is the spontaneous spin-flip rate, Γ is the trion recombination rate and n is the Bose–Einstein occupation number for phonons with energy E equal to the splitting energy. In the fit to the data, we use a density-of-states (shown as a red dotted curve in the Fig. 4e ) centred on the low-energy acoustic phonon line of the inset of Fig. 4a . For comparison, the black dashed curve shows r calculated using a constant spontaneous decay rate. Although a constant spontaneous decay rate explains the behaviour observed in CdSe self-assembled quantum dots [13] , it clearly does not fit our data. The demonstration of stable trion emission via a photo-charging route highlights the role of NC heterostructure engineering in modifying photophysical properties of these materials. This is particularly relevant to NC dynamics, as transitions to the trion state have been held responsible for photoluminescence blinking [40] . This random charge ejection/recombination cycle has even been observed in a recently reported ‘lifetime blinking’ in non-blinking giant NCs [25] . Here we are able to promote the NC to emit solely from its trion state, resulting in ‘true’ non-blinking behaviour; that is continuous emission from a single state of the system. Furthermore, we have shown that both trion charge states and concomitantly their charged biexcitons have high luminescence quantum yields, contrary to observations at room temperature [25] , indicating that Auger recombination is inefficient in these materials. Thus the photo-charging mechanism of our NCs can be attributed to a tunnelling process, which has significant implications for alternative photoluminescence-blinking mechanisms [41] , [42] . Another interesting consequence of NC engineering is revealed in the g -factor measurements. The use of a symmetric zinc-blende crystal lattice enabled us to test the different influences of heavy holes and light holes arising from natural variations in the NC shape. NCs exhibiting four-peaked trion spectra in a magnetic field were identified as corresponding to those with aspect ratios close to unity (spherical), which corresponds to a region of maximal heavy-hole/light-hole mixing. These NCs displayed a remarkable property; approximately isotropic electron and hole g -factors. Thus, we find that spherical zinc-blende NCs effectively overcome the orientation sensitivity of colloidal nanoparticles for which the control of orientation is extremely challenging. We have also demonstrated an exciting property of colloidal NCs that sets them apart from other quantum dots: An acoustic phonon bottleneck that inhibits spin relaxation. This property arises purely due to their finite nanometre size, which results in a low-energy cutoff for acoustic phonon modes. This is the acoustic equivalent to the inhibition of spontaneous emission in cavity quantum electrodynamics, and like its optical equivalent, should promote new research directions with these materials. In particular, the potential to operate at higher magnetic fields without incurring acoustic phonon-induced spin relaxation should be beneficial in stabilizing the spin state against perturbations from environmental nuclei, resulting in longer spin coherence times [15] . Thus, colloidal NCs offer the possibility to considerably extend the operating parameter space for spin-based technologies. The next step will be to study the spin properties of the charged NC ground state. This realization of a long-heralded beneficial finite size effect in single NCs will promote further investigation and open these materials to new applications in quantum information. Synthesis of NCs The CdSe/CdS 4 /ZnS 1 NCs were synthesized via the following steps. Zinc-blende CdSe cores A cadmium oleate (Cd-OA) stock solution was prepared by first degassing 9.3 mmol (1.2 g) of CdO and 106 mmol (30 g) of oleic acid in 120 g of 1-octadecene (ODE) at 100 °C for 30 min [43] . This solution was heated to 300 °C under nitrogen until it became transparent and homogeneous. The Cd-OA solution was then cooled to 100 °C and degassed for a further 30 min to remove any residual water formed during the reaction. The selenium precursor (TOP-Se) was prepared by dissolving 0.47 mmol (0.037 g) of selenium in 3.1 mmol (1.16 g) of trioctylphosphine by sonicating and mixing using a vortex mixer before adding 5.25 g of ODE. The CdSe cores were prepared by rapidly injecting a TOP-Se solution into 7.5 g of the Cd-OA stock solution at 300 °C under nitrogen, after which the temperature was allowed to drop to 230 °C for the growth of crystallites. The growing process was monitored using absorption spectroscopy and the reaction was quenched, by removing it from heat, once the first exciton peak reached 614 nm for a desired QD diameter of 5.25 nm. The QDs were purified using a liquid–liquid extraction process using a combination of methanol, chloroform and acetone to remove excess surfactants. The purified QDs remained in the ODE layer for shelling. CdSe/CdS/ZnS core/shells The graded-seal shelling process was adapted from the successive ion layer adsorption and reaction method [44] . The required amount of washed core particles in ODE was added to a three-necked round bottom flask along with a mixture of ODE/octadecylamine in a 2.5:1 ratio by weight to produce a 40 μM dispersion of NCs. The mixture was degassed at 80 °C for 20 min, pump/purged three times and then heated to 230 °C for shell growth. The calculated amounts of the injection solutions were then added in sequential order beginning with cadmium. Each metal and sulphur injection was allowed to react for 20 and 15 min, respectively. The growth temperature was gradually increased by 5 °C for every metal layer added. Once the final zinc layer was injected, the reaction solution was then annealed at 200 °C for 1 h. The final QD core/shells have 4.5 monolayers of CdS and 1 monolayer of ZnS and are 8.7 nm in diameter. They were again purified using the liquid–liquid extraction technique, and then finally separated from ODE using excess acetone and centrifugation. The resulting pellet was redispersed in toluene for spectroscopy measurements. Cryogenic characterization For cryogenic study, samples were prepared by spin coating clean glass coverslips with approximately nano-molar solutions of NCs into a polymethyl methacrylate matrix. A scanning confocal microscope was used to image single NCs excited with the 532-nm line of a cw frequency-doubled Nd:YAG laser. It is based on a 0.95 numerical aperture objective housed in a magnetic cryostat capable of operation up to 7 T. The sample was mounted on top of a piezoscanner used for raster scanning and for precise NC positioning on the optical axis. The objective axis was perpendicular to the magnetic field, allowing magneto-optical studies in the Voigt configuration. The emitted photons were filtered from the scattered excitation light by a band-pass filter (60 nm full-width at half-maximum) and sent to 30/70 beam splitter that sends the emission to a single photon-counting avalanche photodiode (APD) and a spectrometer (1800, lines per mm grating, focal length 500 mm with a measured spectral resolution of 120 μeV), respectively. Unless otherwise stated, spectra were obtained at 2 K with a pump irradiance of 25 W cm −2 and a 20-s integration time. Single NCs were selected for their spectral and photophysical stability. For the g (2) ( τ ) measurement, the spectrometer was replaced by a second APD with the outputs from both APDs being sent to a time-correlated single photon-counting card, providing both the start and stop pulses. A picosecond-pulsed laser pumps a frequency-doubled optical parametric oscillator to provide a 76 MHz pulse train of ~2 ps pulses at 570 nm. A pulse picker was used to reduce the pulse frequency to 7.6 MHz for the experiment. Residual coincidences involving background photons were negligible in g (2) ( τ ) histograms due to the high signal-to-background ratio. Modelling details The radial wavefunctions plotted in Fig. 1a were obtained by solving the radial wave equation by mapping onto the 1D wave equation via rΨ ( r )→ Ψ′ ( x ). The solutions of the 1D wave equation are trivial, however, the boundary conditions must include Ψ′ (0)=0, as the wavefunction must be finite at the origin. In addition, due to the different charge-carrier effective masses in different regions of the NC, the lowest energy eigenvalue is proportional to u 2 and found as the lowest energy solution to the equation, where m 1 and m 2 are the effective masses of the charge carrier in the regions on either side of the heterojunction. The effective masses and potentials used in the solution were, CdSe: m e =0.13, m hh =0.9, m lh =0.19, V e = V h =0. CdS: m e =0.2, m h =0.8, V e =0.19, V h =0.55. ZnS: m e =0.28, m h =0.57, V e =0.9, V h =0.9. Ligand shell: m e = m h =1, V e = V h =10. The exciton fine structure for CdSe NCs with a zinc-blende crystal structure was adapted from the theory of Efros et al. [35] by neglecting the crystal field splitting term and substituting the band-edge effective mass parameters appropriate for the zinc-blende structure [45] . The eigenvalue solutions are modified to express them in terms of the aspect ratio for ellipsoidal perturbations for a constant radius parameter, a . To estimate the energy of the lowest l =2 acoustic phonon mode, in a composite core/shell NC, we use the estimates of the core size (5.3 nm) and total NC size (10 nm) to calculate the ratio of the core to shell material. Considering only the CdSe core and the CdS shell, the NC comprises ~85% shell, so the longitudinal sound velocity is estimated as a weighted average of v L =3559, m s −1 and 4289, m s −1 for CdSe and CdS, respectively. The l =2 mode frequency is then calculated according to, where R is the radius. Identification of the acoustic phonon peaks is also conducted in a fashion that is independent of the NC size and absolute elastic properties, assuming only that the ratio of the longitudinal to transverse sound velocities remains constant. The material properties of CdSe and CdS are such that the ratio of the longitudinal to transverse sound velocities is nearly equivalent in the bulk materials [46] . This means the solutions for the acoustic phonon energies will have a common scaling factor. Thus, we can write the size-dependent energy for the following three acoustic phonon modes as, representing the first two l =2 modes and the l =0 breathing mode, respectively. Any ratio of these energy solutions will be independent of the NC size and material properties, providing a robust fingerprint of the mode structure, which is used to identify the acoustic phonons observed in Fig. 4a . The density-of-states function used in fitting the rate equation model (equation 1) to the acoustic phonon bottleneck data was approximated by a Voigt function centred on the l =2 acoustic phonon energy (650 μeV). A good fit was only possible with a small Lorentzian width of 2 μeV and a 120 μeV Gaussian width. How to cite this article: Fernée, M.J. et al. Magneto-optical properties of trions in non-blinking charged nanocrystals reveal an acoustic phonon bottleneck. Nat. Commun. 3:1287 doi: 10.1038/ncomms2300 (2012).